Population structure analysis and laboratory monitoring ofShigellaby core-genome multilocus sequence typing The laboratory surveillance of bacillary dysentery is based on a standardised Shigella typing scheme that classifies Shigella strains into four serogroups and more than 50 serotypes on the basis of biochemical tests and lipopolysaccharide O-antigen serotyping. Real-time genomic surveillance of Shigella infections has been implemented in several countries, but without the use of a standardised typing scheme. Here, we study over 4000 reference strains and clinical isolates of Shigella , covering all serotypes, with both the current serotyping scheme and the standardised EnteroBase core-genome multilocus sequence typing scheme (cgMLST). The Shigella genomes are grouped into eight phylogenetically distinct clusters, within the E. coli species. The cgMLST hierarchical clustering (HC) analysis at different levels of resolution (HC2000 to HC400) recognises the natural population structure of Shigella . By contrast, the serotyping scheme is affected by horizontal gene transfer, leading to a conflation of genetically unrelated Shigella strains and a separation of genetically related strains. The use of this cgMLST scheme will facilitate the transition from traditional phenotypic typing to routine whole-genome sequencing for the laboratory surveillance of Shigella infections. Shigella belongs to the Enterobacteriaceae family, and causes bacillary dysentery, a common cause of diarrhoea in low- and middle-income countries. It has been estimated that this intracellular human pathogen, which is transmitted via the faecal-oral route with a very low infectious dose (10–100 cells), is responsible for over 210,000 deaths per year, mostly in children under the age of 5 years [1] , [2] , [3] . In high-income countries, Shigella infections also occur in travellers and in some high-risk groups, such as men who have sex with men (MSM) and Orthodox Jewish communities [2] , [3] , [4] , [5] . The morbidity of these infections is currently increasing due to growing resistance to antimicrobial drugs in these bacteria [2] , [3] , [5] , [6] . Since 2016, highly drug-resistant (i.e., resistant to at least ciprofloxacin, azithromycin and third-generation cephalosporins) S. sonnei isolates have been found in the US, England and Australia [3] . Laboratory surveillance of Shigella infections was initiated several decades ago, and was facilitated by the adoption of a standardised Shigella typing scheme in the late 1940s [7] . This scheme, which is still in use today, is based on biochemical tests and serotyping (slide agglutination with typing sera directed against the different Shigella lipopolysaccharide O-antigens). It splits the Shigella genus into four serogroups (originally considered to be species): Shigella dysenteriae , S. boydii , S. flexneri and S. sonnei ; these four serogroups are then subdivided into more than 50 serotypes. However, modern population genetics methods based on bacterial DNA sequences, such as multilocus sequence typing (MLST) analysis (which analyses the allelic profiles of — generally seven — housekeeping genes), and, more recently, core-genome single-nucleotide variant (cgSNV) analysis, have shown that shigellae form distinct lineages within the species E. coli , from which they emerged following the acquisition of a large virulence plasmid (VP) enabling the bacterium to invade intestinal cells [8] , [9] , [10] , [11] . In parallel, these host-restricted pathogens converged independently on the Shigella phenotype (non-motility, no decarboxylation of lysine, no use of citrate and malonate, and other characteristics, as reported by Pupo and coworkers [8] ) through genome degradation. More recent molecular approaches have shown that the current standardised Shigella typing scheme does not accurately reflect the population structure of this pathogen [8] . However, some molecular data have been taken into account in an update of the Shigella serotyping scheme. S. boydii serotype 13, for example, was withdrawn from the classification, because it was shown to belong to another species, Escherichia albertii , and lacked the VP [12] , [13] . In an increasing number of countries, the laboratory surveillance of Shigella infections has now passed from conventional serotyping to real-time genomic surveillance [10] , [14] . The genomic methods used mostly target the O-antigen gene cluster ( rfb ) or the S. flexneri serotype-converting prophages, to ensure serotype specificity [14] , [15] . In addition, a set of 22 accessory genome genes was recently used to reassign Shigella serotypes to eight clusters [16] . Whilst these methods maintain backward compatibility between the genomic and serotyping data, they do not fully exploit the full resolution of genomic data. Hence, an extension of the MLST method to cover hundreds to thousands of core-genome genes has been developed. This high-resolution method, core-genome MLST (cgMLST), has been successfully used in the surveillance of many pathogens, including Listeria monocytogenes [17] and Salmonella enterica [18] . Furthermore, cgMLST data are easy to interpret with clustering threshold methods, such as the hierarchical clustering (HierCC) [19] implemented in EnteroBase [18] , [19] . However, until now, cgMLST has never been used for the comprehensive description of Shigella populations, and the utility of this method for the genomic surveillance of Shigella infections has not previously been assessed. In this study, we analyse over 4000 genomes from phenotypically characterised Shigella strains representative of the global diversity of this pathogen. We aimed: (i) to resolve the population structure of Shigella using cgMLST, (ii) to create a dictionary of correspondence between cgMLST HC and serotyping data, (iii) to evaluate the performance of different in silico serotype prediction tools and (iv) to update the Shigella serotyping scheme by describing new serotypes. We demonstrate that the combination of cgMLST HC with rfb gene cluster analysis would enhance the laboratory surveillance of Shigella infections, while maintaining backward compatibility with the current serotyping scheme. Global population structure of S higella We assembled and sequenced a collection of 317 Shigella strains chosen on the basis of their representativeness of the known diversity of Shigella populations (i.e., covering all serogroups and serotypes, and the different lineages or phylogroups of S. sonnei and S. flexneri ). The genomic diversity of this “reference” dataset was further increased by adding another 81 publicly available Shigella genomes (these 81 genomes representing the “reference+” dataset). The 398 genomes studied were from strains belonging to the S. flexneri ( n = 191), S. dysenteriae ( n = 83), S. boydii ( n = 80) and S. sonnei ( n = 44) serogroups (Supplementary Table 4 ). We determined the wider phylogenetic context of these Shigella genomes by also analysing 95 E. coli genomes, including 27 EIEC from eight different EIEC genomic clusters and 68 (of the 72) strains from the ECOR collection, considered representative of the diversity of natural populations of E. coli [20] . We studied these 493 genomes by two different approaches: cgMLST and SNV-based clustering. 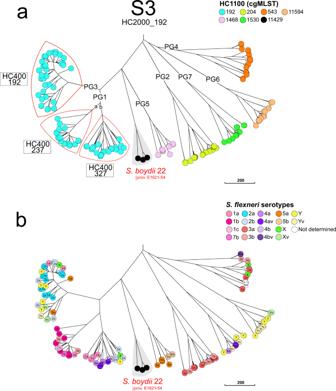Fig. 4: A NINJA NJ GrapeTree showing the population structure of theShigellaS3 cluster (HC2000_192). This subtree is based on the tree shown in Fig.1.aThe tree nodes are colour-coded by HC1100 data. TheS. flexneriphylogenetic groups (PG) identified by Connor and coworkers2are indicated. Some HC400 clusters are indicated to separate PG3 from PG1.S. boydi22 (formerly prov. E1621-54) is shown.bThe tree nodes are colour-coded byS. flexneriserotype. The scale bar indicates the number of cgMLST allelic differences. We used the EnteroBase Escherichia / Shigella cgMLST (2513 genes) scheme, which also assigns bacterial genomes to single-linkage hierarchical clusters (HCs) in real-time, at 13 fixed levels of resolution, ranging from HC0 (high-resolution clusters consisting of identical genomes with no allelic differences) to HC2350 (low-resolution clusters consisting of genomes with up to 2350 allelic differences). A previous evaluation by Zhou and coworkers [19] found that in the genus Escherichia , cluster assignments at the HC2350, HC2000-HC1500, and HC1100 levels could be used to distinguish species, super-lineages and ST complexes, respectively. Since these levels of resolution are appropriate for routine surveillance, we predominantly used cgMLST HC2000 to HC400 levels to define the naturally, genetically discrete populations of Shigella (Fig. 1 and Supplementary Fig. 1 ). Fig. 1: Population structure of Shigella spp. based on the cgMLST allelic differences between 493 Shigella and E. coli reference genomes. a A NINJA neighbour-joining (NJ) GrapeTree with tree nodes colour-coded by Shigella serogroup and E. coli pathovar. b A NINJA NJ GrapeTree with tree nodes colour-coded by HC2000 data. HC2000 clusters with fewer than two isolates are represented by white nodes. The different Shigella cgMLST clusters are labelled. For the SON cluster, the different genomic lineages of S. sonnei are indicated with Latin numerals. For the S. flexneri serotypes in cluster S3, the phylogenetic groups (PG1 to PG7) identified by Connor and coworkers [2] are also indicated. The scale bar indicates the number of cgMLST allelic differences. The interactive version of the tree is publicly available from http://enterobase.warwick.ac.uk/ms_tree?tree_id=55118 and http://microreact.org/project/kP4HJjriDvAfTS4Ed3Avx8/01568b6f . Full size image Accordingly, by cgMLST, all 493 genomes belonged to the same HC2350 cluster (HC2350_1) defining the species Escherichia coli (Supplementary Data 1 ). As expected, all the Shigella and EIEC genomes contained the pathogenicity gene ipaH , whereas the ECOR genomes did not (Supplementary Fig. 2 ). A NINJA neighbour-joining (NJ) tree of core genomic allelic distances was generated with the dataset for the 493 Shigella and E. coli genomes (Fig. 1a ). The differential contribution of the reference and reference+ datasets to Shigella population diversity is shown in Supplementary Fig. 2 . Visual examination of the colour-coded HC2000 tree revealed that the Shigella genomes were grouped into eight different HC2000 clusters (Fig. 1b ). Seven of these HC2000 clusters contained exclusively Shigella genomes. The eighth, HC2000_2, contained S. dysenteriae type 8 and E. coli (EIEC and ECOR) genomes. Four HC2000 clusters contained Shigella genomes from a single serotype: HC2000_305 ( S. sonnei ), HC2000_1463 ( S. dysenteriae type 1), HC2000_44944 ( S. dysenteriae 10), and HC2000_45542 ( S. boydii 12). These clusters are referred to as SON, SD1, SD10 and SB12, respectively. Three clusters comprised multiple serogroups and serotypes: HC2000_1465, HC2000_4118, and HC2000_192, referred to as S1, S2 and S3, respectively (Fig. 2 – 4 , Supplementary Notes sections “Genomic clustering of Shigella reference strains” and “Discrepancies with published studies”). Fig. 2: A NINJA NJ GrapeTree showing the population structure of the Shigella S1 cluster (HC2000_1465). This subtree is based on the tree shown in Fig. 1 . The tree nodes are colour-coded by serogroup. The numbers within nodes indicate the serotype. HC1100 designation is indicated next to each subcluster. Novel and provisional (prov.) Shigella serotypes are also shown. NST non-serotypeable. The scale bar indicates the number of cgMLST allelic differences. Full size image Fig. 3: A NINJA NJ GrapeTree showing the population structure of the Shigella S2 cluster (HC2000_4118). This subtree is based on the tree shown in Fig. 1 . The tree nodes are colour-coded by serogroup. The numbers within nodes indicate the serotype. HC1100 designation is indicated next to each subcluster. Provisional (prov.) Shigella serotypes are also shown. The scale bar indicates the number of cgMLST allelic differences. Full size image Fig. 4: A NINJA NJ GrapeTree showing the population structure of the Shigella S3 cluster (HC2000_192). This subtree is based on the tree shown in Fig. 1 . a The tree nodes are colour-coded by HC1100 data. The S. flexneri phylogenetic groups (PG) identified by Connor and coworkers [2] are indicated. Some HC400 clusters are indicated to separate PG3 from PG1. S. boydi 22 (formerly prov. E1621-54) is shown. b The tree nodes are colour-coded by S. flexneri serotype. The scale bar indicates the number of cgMLST allelic differences. Full size image The HC2000 clusters could themselves be divided into five or more HC1100 subclusters (S1a-S1e, S2a-S2f and PG1-PG7). 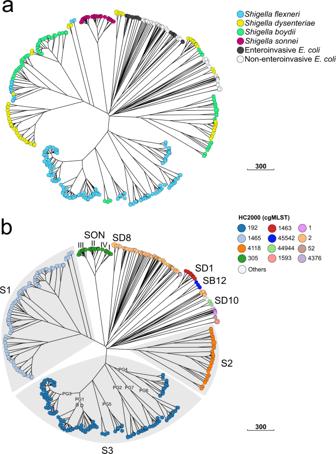Of note, identical serotypes were found in different clusters and subclusters. Fig. 1: Population structure ofShigellaspp. based on the cgMLST allelic differences between 493ShigellaandE. colireference genomes. aA NINJA neighbour-joining (NJ) GrapeTree with tree nodes colour-coded byShigellaserogroup andE. colipathovar.bA NINJA NJ GrapeTree with tree nodes colour-coded by HC2000 data. HC2000 clusters with fewer than two isolates are represented by white nodes. The differentShigellacgMLST clusters are labelled. For the SON cluster, the different genomic lineages ofS. sonneiare indicated with Latin numerals. For theS. flexneriserotypes in cluster S3, the phylogenetic groups (PG1 to PG7) identified by Connor and coworkers2are also indicated. The scale bar indicates the number of cgMLST allelic differences. The interactive version of the tree is publicly available fromhttp://enterobase.warwick.ac.uk/ms_tree?tree_id=55118andhttp://microreact.org/project/kP4HJjriDvAfTS4Ed3Avx8/01568b6f. For example, S. boydii 11 was found in S1b and S2c, S. dysenteriae 3 in S1a and S1b, and S. flexneri 6 in S1b and S1e (Table 1 ). Our analysis extends a polyphyletic nature to the majority of S. flexneri serotypes and subserotypes, found in S3 (Fig. 4 ). Each of these six HC1100 subclusters of S3 contained two or more S. flexneri serotypes, with identical serotypes found in different subclusters (Fig. 4b and Table 1 ). At a higher level of resolution, 10 Shigella serotypes were grouped within specific HC400 clusters, whereas the other serotypes remained mixed in HC400 clusters or split between two to seven HC400 clusters (Table 1 ). However, with HC1100 and HC400, we found, for S3, a correspondence between the clustering obtained with cgMLST and that obtained by Connor and coworkers [2] , who previously subdivided S. flexneri 1–5, X, Y into seven phylogenetic groups (PG1-PG7), based on a Bayesian analysis of population structure (Fig. 4a , Supplementary Notes section “Genomic clustering of Shigella reference strains”). Finally, we confirmed that biochemically atypical S. boydii 14 (aerogenic) and S. dysenteriae 3 (aerogenic and mannitol positive) strains [21] , [22] – the status of which remained a matter of debate for decades – were genuine Shigella strains belonging to S1b ( Supplementary Notes section “Aerogenic strains of S. boydii 14 and S. dysenteriae 3”). The atypical S. dysenteriae 3 strain was derived from a S. flexneri 6 strain following the acquisition of the S. dysenteriae 3 rfb gene cluster (see next section “Genomic analysis of the O-antigen gene cluster”). Table 1 Distribution of the different Shigella serotypes in clusters S1, S2, and S3 of 398 Shigella reference and reference+ genomes according to their HC2000, HC1100, and HC400 data. Full size table We evaluated the accuracy of low-resolution cgMLST HCs for grouping Shigella genomes into different clusters of phylogenetic significance by employing another approach. We used the same dataset of 493 Shigella and E. coli genomes to infer two SNV-based ML trees: one based on 92,688 SNV sites (including recombinant sites) and the second on 5129 recombination-free SNVs. We compared these SNV-based clusterings (with strong bootstrap support) to clusters inferred by cgMLST HC. We found that the clustering of Shigella populations by HC2000 and by HC1100 were congruent with both core-genome SNV phylogenies (Fig. 5 and Supplementary Fig. 3 ). Even though cgMLST allelic distances (based on allelic changes counted as single genetic events, regardless of the number of SNVs involved) are reliable indicators of population structure, especially for routine surveillance tasks, SNVs are generally preferred for more detailed studies including long-term evolutionary dynamics. This likely accounts for the topological differences in the deep structures of cgSNV and cgMLST phylogenetic trees (Figs. 1 and 5 and Supplementary Fig. 3 ). Since the focus of this study was the use of cgMLST for routine surveillance of Shigella infections, resolution of these ancestral differences was not investigated further. Fig. 5: Population structure of 493 Shigella and E. coli reference genomes based on core-genome SNVs. This maximum-likelihood phylogenetic tree genomes are based on 92,688 core-genome single-nucleotide variants (SNVs). Nodes supported by bootstrap values ≥95% are indicated by red dots. Phylogenetic clades containing Shigella genomes are labelled with the same nomenclature (S1-S3, SON, SD1, SD8, SD10, and SB12) as in Fig. 1 . All the Shigella genomes are also labelled on the right with cgMLST HC2000 and HC1100 data. The scale bar indicates the number of nucleotide substitutions per variable sites (SNVs). Full size image For confirmation of the robustness of the population structure of Shigella established by cgMLST analysis of our reference datasets, we also applied cgMLST to 3870 clinical Shigella isolates received by the FNRC-ESS between 2017 and 2020 (the “routine” dataset), in the framework of the French national surveillance programme for Shigella infections (see the methods section “Strain selection and typing”). All these isolates were characterised phenotypically, on the basis of biochemical reactions and serotyping. They belonged to S. dysenteriae ( n = 53), S. boydii ( n = 101), S. flexneri ( n = 1555) and S. sonnei ( n = 2161). All but one of these 3870 genomes were assigned to known serotype/HC2000/HC1100/HC400 combinations, without inconsistencies (Supplementary Data 1 and Supplementary Fig. 4 ). The exception was an HC1100_204 (PG2) S. flexneri isolate, grouped into a new HC400 cluster, HC400_11853. The stability of the cgMLST data was assessed by comparing allelic differences between pairs of Shigella isolates recovered from the same patient within months of each other (Supplementary Table 5 ). The routine isolates included 34 such pairs of isolates, each recovered from a single patient within 90 days (mean interval of 12 days between samplings). 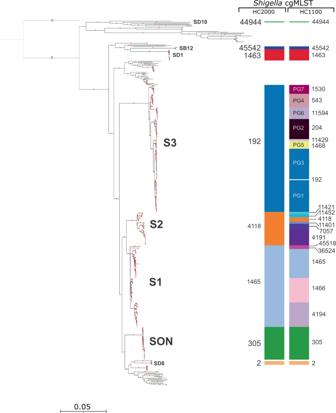Fig. 5: Population structure of 493ShigellaandE. colireference genomes based on core-genome SNVs. This maximum-likelihood phylogenetic tree genomes are based on 92,688 core-genome single-nucleotide variants (SNVs). Nodes supported by bootstrap values ≥95% are indicated by red dots. Phylogenetic clades containingShigellagenomes are labelled with the same nomenclature (S1-S3, SON, SD1, SD8, SD10, and SB12) as in Fig.1. All theShigellagenomes are also labelled on the right with cgMLST HC2000 and HC1100 data. The scale bar indicates the number of nucleotide substitutions per variable sites (SNVs). These pairs displayed between 0 and 5 (mean 1.5) cgMLST differences, for the 2513 alleles tested. Genomic analysis of the O-antigen gene cluster The current typing scheme is mostly based on serotyping (targeting the variability of the O antigen, the polysaccharide part of lipopolysaccharide (LPS), the major bacterial surface antigen) and certain metabolic markers ( Supplementary Notes “Genomic analysis of metabolic markers used in the current Shigella typing scheme”). The Shigella O antigen gene cluster ( rfb ) is located on the chromosome, except in S. sonnei , in which it is located on a plasmid. The size of these rfb clusters ranges from 9 kb to 17 kb [23] . Consistent with their phylogenetic relationships, the rfb clusters of Shigella serotypes are identical, highly similar to, or adapted from E. coli O-antigen gene clusters, accounting for the many cross-agglutinations observed with the serotyping scheme [23] . We extended this analysis to populations not previously considered (Fig. 6 ) and showed that similarity between E. coli and Shigella rfb DNA sequences was also identified in S. dysenteriae 8 and E. coli O38, and in S. boydii 22 (formerly S. boydii provisional (prov.) E1621-54, see next section “Updating the Shigella typing scheme”) and E. coli O7 (Fig. 7 ). For both these Shigella serotypes, cross-agglutination with the corresponding E. coli serotypes was previously reported by Ewing [24] . Finally, the rfb from a new serotype, S. dysenteriae 16, originated from another species of Escherichia , E. albertii (serotype O2). Our genomic analysis also revealed very closely related rfb clusters present in the Shigella strains belonging to polyphyletic serotypes: identities of 13,192/13,622 (97%), gaps 3/13,622 (0%) between the S. boydii 11 S1b and S2c rfb gene clusters; and identities of 12,800/12,825 (99%) with no gap between the S. dysenteriae 3 S1a and S1b rfb gene clusters; identities of 10,431/10,448 (99%) with no gap between the S. flexneri 6 S1b and S1e rfb gene clusters. Fig. 6: Representation of all previously and newly characterised Shigella O-antigen gene clusters. The names underlined correspond to those presented for the first time. Open arrows represent the location and orientation of putative genes. SS a is a chromosomal remnant rfb from S. sonnei . A b in superscript indicates that the cluster is located on a plasmid. A 1 in superscript indicates that the gene may be truncated by an IS 1 in some strains. Full size image Fig. 7: Phylogenetic tree for all Shigella and E. coli O-antigen gene clusters. The Shigella O-antigen gene clusters ( rfb ) characterised in this study are indicated by an asterisk. Nodes supported by bootstrap values ≥95% are indicated by red dots. S. boydii rfb genes are shown in green, S . dysenteriae rfb genes are shown in orange, S. flexneri rfb genes are shown in blue, and S. sonnei rfb genes are shown in red. The scale bar indicates the number of nucleotide substitutions per variable sites. Full size image Updating the Shigella typing scheme In recent decades, several provisional new serotypes of S. dysenteriae and S. boydii have been suggested [25] , [26] . However, the phylogenetic relationships between these different provisional serotypes have not been investigated. We characterised these relationships in detail ( Supplementary Notes section “Updating the Shigella typing scheme”). We found that these provisional serotypes all belonged to the three main Shigella clusters, S1 to S3 (Fig. 2 – 4 ), and that many of those reported under different names were actually identical. After curation, the provisional serotypes found to belong to new serotypes were named S. dysenteriae 16–18, S. boydii 21 and S. boydii 22, and we propose to add them to the official serotyping scheme. All new Shigella serotypes possessed rfb clusters, similar to those found in known E. coli or E. albertii serotypes. All the reference strains for these new serotypes are now available from the Collection de l’ Institut Pasteur (CIP) or the National Collection of Type Cultures (NCTC). However, for S. dysenteriae prov. BEDP 02-5104, we propose to retain a provisional status, as our analysis ( Supplementary Notes section “Updating the Shigella typing scheme”) suggests that this serotype is probably a S. dysenteriae 2 strain that has acquired an O-antigen-modifying plasmid from E. coli or Citrobacter , the expression of which has replaced the expression of the chromosomal genes. This plasmid also carries a raffinose operon, accounting for the use of this trisaccharide by S. dysenteriae prov. BEDP 02-5104, a very unusual trait in S. dysenteriae [26] . Performance of available in silico serotype prediction tools In silico serotyping tools have been developed by various groups, and can be used to maintain links with the current Shigella serotyping system. We assessed the performances of the three tools currently available: the “SeroPred” tool [18] (implemented in EnteroBase), ShigaTyper [14] (using a short-read mapping approach), and ShigEiFinder [16] (using either short reads or assemblies) with our 316 reference strain genomes with known serotype designations (Supplementary Tables 4 , 6 and 7 ). When all Shigella serotypes and subserotypes were considered (SeroPred does not discriminate the serotypes and subserotypes of S. flexneri 1–5, X and Y), the rates of correct assignment were 80.1% (253/316), 84.5% (267/316) and 83.9% (265/316) for ShigaTyper, ShigEiFinder (short reads) and ShigEiFinder (assemblies), respectively. ShigEiFinder gave the best serotype prediction results, whether based on short reads or assemblies, particularly for S. sonnei and S. boydii (Fig. 8 and Supplementary Table 6 ). However, 100% of the strains belonging to S. boydii 10 and to the new serotypes S. dysenteriae 17 and S. boydii 21, and 14–20% of the strains from S. boydii 11, S. boydii 14 and S. dysenteriae 2 were incorrectly assigned by ShigEiFinder. 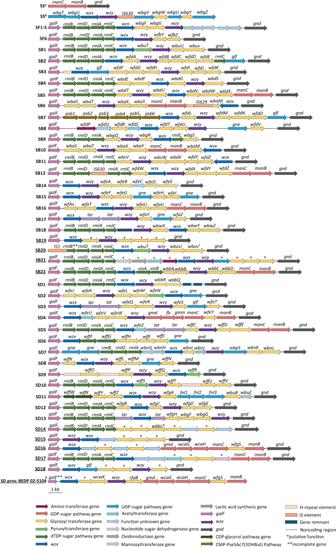Fig. 6: Representation of all previously and newly characterisedShigellaO-antigen gene clusters. The names underlined correspond to those presented for the first time. Open arrows represent the location and orientation of putative genes. SSais a chromosomal remnantrfbfromS. sonnei. A b in superscript indicates that the cluster is located on a plasmid. A 1 in superscript indicates that the gene may be truncated by an IS1in some strains. Furthermore, all the genomes belonging to S. dysenteriae prov. BEDP 02-5104 were incorrectly predicted to be S. dysenteriae 2, while 83% of the strains from the new serotype S. dysenteriae 16 were incorrectly predicted to be S. dysenteriae prov. 96–265, and 17% were not assigned. Fig. 8: Graphical representation of the in silico serotyping results for 316 Shigella reference strains according to each serotype prediction tool. Stacked-bar chart displaying the results (percentage assignment) per tool for each Shigella serotype. E, the SeroPred tool implemented in EnteroBase [18] ; T, ShigaTyper [14] ; R, ShigEiFinder [16] using short reads; F, ShigEiFinder using SPAdes assemblies. SB S. boydii , SD S. dysenteriae , SON S. sonnei , SF S. flexneri . A correct assignment means that the predicted serotype was the same as the phenotypically determined serotype. An uncertain assignment means that the correct serotype was listed among others or, for ShigEiFinder that only the cluster level (Cs1 to Cs3) was obtained. An incorrect assignment means that the predicted serotype was different from the phenotypically determined serotype. “None” means that no serotype was predicted. More detailed results can be found in Supplementary Table 6 . Full size image When analysing the 3861 “routine” genomes from isolates with known serotype designations (9/3870 could not be serotyped, Supplementary Table 4 ), 96.2% (3713/3861), 55.9% (2157/3861) and 80.8% (3120/3861) of the strains were correctly assigned by ShigaTyper, ShigEiFinder (short reads) and ShigEiFinder (assemblies), respectively. ShigEiFinder performed less well than ShigaTyper with this routine dataset (Fig. 9 and Supplementary Table 7 ). In particular, most of the results obtained with short reads were “uncertain” (i.e., assignment to a Shigella cluster, but not to a serotype). 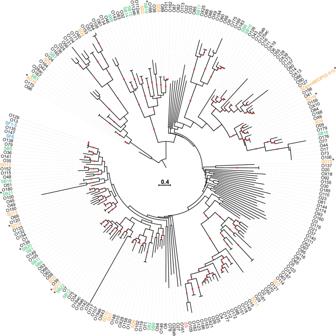Fig. 7: Phylogenetic tree for allShigellaandE. coliO-antigen gene clusters. TheShigellaO-antigen gene clusters (rfb) characterised in this study are indicated by an asterisk. Nodes supported by bootstrap values ≥95% are indicated by red dots.S. boydii rfbgenes are shown in green, S. dysenteriae rfbgenes are shown in orange,S. flexneri rfbgenes are shown in blue, andS. sonnei rfbgenes are shown in red. The scale bar indicates the number of nucleotide substitutions per variable sites. ShigEiFinder uses 22 accessory genome (non-O antigen) genes to assign Shigella genomes to eight clusters, with the serotype assignment based on the Shigella serotype-specific wzx / wzy genes (and O-antigen modification genes for S. flexneri ). The inferior performance of ShigEiFinder can be explained by the low read coverage of the AT-rich rfb gene cluster for the “routine” genomes. Our public health sequencing platform (P2M) uses the Nextera XT kit (Illumina, San Diego, CA, USA), according to an in-house protocol, for library preparation, and transposase-based library generation is known to be biased against AT-rich sequences [14] . Fig. 9: Graphical representation of the in silico serotyping results for 3861 Shigella “routine” isolates according to each serotype prediction tool. Stacked-bar chart displaying the results (percentage assignment) per tool for each Shigella serotype. E, the SeroPred tool implemented in EnteroBase [18] ; T, ShigaTyper [14] ; R, ShigEiFinder [16] using short reads; F, ShigEiFinder using SPAdes assemblies. SB S. boydii , SD S. dysenteriae , SON S. sonnei , SF S. flexneri . A correct assignment means that the predicted serotype was the same as the phenotypically determined serotype. An uncertain assignment means that the correct serotype was listed among others or for ShigEiFinder that only the cluster level (Cs1 to Cs3) was obtained. An incorrect assignment means that the predicted serotype was different from the phenotypically determined serotype. “None” means that no serotype was predicted. More detailed results can be found in Supplementary Table 7 . Full size image We present here a broad overview of the population of Shigella . The hierarchical clustering of cgMLST data and a cgSNV analysis showed that Shigella strains belong to eight phylogenetically distinct clusters within the E. coli species. Our results are consistent with previous studies suggesting multiple origins of the “ Shigella ” phenotype [8] , [27] . However, the higher resolution of cgMLST and comprehensive sampling from thousands of phenotypically characterised isolates and reference strains covering all serotypes – including provisional serotypes and atypical strains – made it possible to complete, and in some cases amend, the Shigella population structure obtained in previous studies. The 70-year-old Shigella typing scheme, which is still in use today, was based on biochemical characteristics, antigenic relationships, and tradition [7] . We show here that, unlike cgMLST, this scheme does not reflect the natural population structure of these bacteria. In particular, the Shigella serogroups/species are artificial constructs developed from data for antigen and metabolic markers affected by IS element inactivation or horizontal gene transfer. The presence and expansion of large numbers of ISs in Shigella genomes can disrupt coding sequences or cause genome rearrangements and deletions, thereby altering the nature of both the O-antigen and the rare phenotypic markers identified in this bacterium with weak metabolic activity [9] . For example, S. boydii 6 and 20 arose in subcluster 1c following the insertion of a single IS within the rfb cluster of S. boydii 10 and 1, respectively. Serotype diversification, which is observed mostly in clusters S1 to S3, also occurs via horizontal gene transfer of the O-antigen-encoding rfb cluster from Escherichia or Shigella donors [8] , [28] . Horizontal gene transfer outside of the rfb cluster can also alter the serotype of a strain, as illustrated particularly clearly by the S3 cluster. All the S. flexneri strains in this cluster share the same O-antigen backbone structure, and their serotypes are determined by glucosylation and/or O-acetylation modifications to the O-antigen tetrasaccharide repeat, conferred by prophage-encoded gtr and/or oac genes, respectively [15] . Plasmid-mediated serotype conversion by the O-antigen phosphoethanolamine transferase gene ( opt ) has also been reported in S. flexneri [15] . Each of the seven S. flexneri phylogenetic groups (PGs) described by Connor and coworkers [2] , based on a cgSNV analysis, contained two or more of these serotypes. This serotyping method does not reflect the genetic relatedness between Shigella isolates, and has a number of other disadvantages, including being time-consuming, having intra- and interspecies cross-reactivity, not allowing for typing of rough strains and new serotypes [14] , [25] . Therefore, modern laboratory surveillance of Shigella infections should now be based on phylogenetically relevant methods rather than simply on molecular or in silico serotyping [10] , [14] , [15] , [16] . The cgMLST HC analysis provides, in a single step, a wide range of fixed clustering levels, from HC0 (no allelic differences allowed) to HC2350 (maximum of 2350 allelic differences allowed), with a standard and stable nomenclature. In our study, cgMLST HC analysis at low levels of resolution (HC2000 to HC400) provided sufficient resolution to monitor the trends in globally circulating Shigella types. The different clusters of S higella can be identified with HC2000. Using HC1100 and, in certain instances HC400, can provide added detail needed to reveal additional subclusters. This is particularly interesting for S3, which contains the S. flexneri 1–5, X, and Y serotypes generated via horizontal gene transfer rather than by vertical descent. We therefore recommend integrating the seven phylogenetic groups (PG1-PG7) described for S. flexneri into routine genomic surveillance for S. flexneri . These PGs can be easily inferred from cgMLST HC1000/HC400; it is even possible to obtain up to eight groups (after subdividing PG1 into PG1a and PG1b). High-resolution subtyping (at strain level) is needed for the most frequent — and often genetically homogeneous — Shigella serotypes, such as S. sonnei and S. flexneri 2a, for the identification of a single-source outbreak or to follow up an epidemic strain. Such studies have traditionally employed cgSNV analysis [4] , [6] . 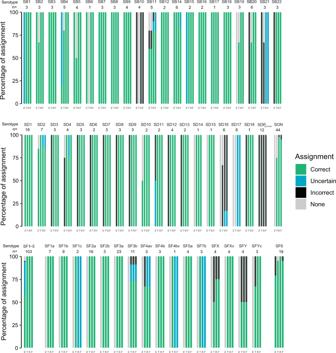Fig. 8: Graphical representation of the in silico serotyping results for 316Shigellareference strains according to each serotype prediction tool. Stacked-bar chart displaying the results (percentage assignment) per tool for eachShigellaserotype. E, the SeroPred tool implemented in EnteroBase18; T, ShigaTyper14; R, ShigEiFinder16using short reads; F, ShigEiFinder using SPAdes assemblies. SBS. boydii, SDS. dysenteriae, SONS. sonnei, SFS. flexneri. A correct assignment means that the predicted serotype was the same as the phenotypically determined serotype. An uncertain assignment means that the correct serotype was listed among others or, for ShigEiFinder that only the cluster level (Cs1 to Cs3) was obtained. An incorrect assignment means that the predicted serotype was different from the phenotypically determined serotype. “None” means that no serotype was predicted. More detailed results can be found in Supplementary Table6. 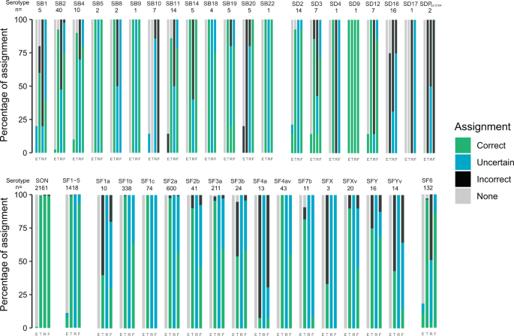Fig. 9: Graphical representation of the in silico serotyping results for 3861Shigella“routine” isolates according to each serotype prediction tool. Stacked-bar chart displaying the results (percentage assignment) per tool for eachShigellaserotype. E, the SeroPred tool implemented in EnteroBase18; T, ShigaTyper14; R, ShigEiFinder16using short reads; F, ShigEiFinder using SPAdes assemblies. SBS. boydii, SDS. dysenteriae, SONS. sonnei, SFS. flexneri. A correct assignment means that the predicted serotype was the same as the phenotypically determined serotype. An uncertain assignment means that the correct serotype was listed among others or for ShigEiFinder that only the cluster level (Cs1 to Cs3) was obtained. An incorrect assignment means that the predicted serotype was different from the phenotypically determined serotype. “None” means that no serotype was predicted. More detailed results can be found in Supplementary Table7. The high-resolution levels of EnteroBase cgMLST, HC5 and HC10, have been used to detect foodborne outbreaks caused by Salmonella [18] , [29] , [30] and enterohaemorragic E. coli [31] . Our study aimed to assess the EnteroBase cgMLST tool as a replacement for the current serotyping scheme. However, this study did not set out to assess the performance of HC5 and HC10 for the high-resolution subtyping of prevalent Shigella populations. For these purposes, a robust and practical hierarchical SNV-based genotyping scheme developed for S. sonnei by Hawkey and coworkers [3] provided more resolution than even the high-resolution levels of EnteroBase cgMLST. For example, unlike the hierarchical SNV-based genotyping scheme, HC5 (and even HC10) could not easily identify the internationally recognised S. sonnei epidemic strains, such as those resistant or highly resistant to multiple drugs that have recently spread among MSM globally. These epidemic strains were split into multiple HC5 and HC10 clusters with non-informative numbers, in contrast to the findings with the SNV-based genotyping scheme (which indicates the lineage, clade, subclade, and, when necessary, higher-resolution genotypes and strains of epidemiological interest, with a human-readable alias; e.g., 3.6.1.1.2 (CipR.MSM5)). Despite the utility of our proposed EnteroBase cgMLST-based approach in routine surveillance, it has clear limitations for the global surveillance of S. sonnei infections. Despite the aforementioned limitations in select circumstances, the use of such standardised cgMLST HC data makes it possible to query EnteroBase, which contains over 160,000 E. coli /S higella genomes, to identify strains with similar HC types at any level of resolution. This can facilitate the investigation of unusual types of Shigella (e.g., our analysis of the provisional serotypes) or outbreaks with an international dimension [32] . Importantly, the use of cgMLST HC data in surveillance should be paired with in silico serotyping to achieve backward compatibility with the current serotyping scheme. This is crucial for the maintenance of international surveillance with laboratories that cannot currently afford genomic surveillance and to prevent disjunction with the seven decades of serotyping data accumulated worldwide. To this end, we found that ShigaTyper [14] and ShigEiFinder [16] were promising tools. However, both require optimisation in the choice of molecular targets for certain serotypes. The complete set of rfb sequences provided by our study would be helpful for improving them. ShigEiFinder also requires optimisation of the read mapping thresholds used to determine the presence or absence of the O-antigen genes. In conclusion, by studying >4000 serotyped reference strains and routine isolates covering the overall diversity of Shigella , we were able to demonstrate that cgMLST is a robust and portable genomic method revealing natural populations for this pathovar of E. coli . The cgMLST method has substantial added value in the framework of the laboratory monitoring of Shigella , as it prevents genetically unrelated strains from being conflated, and genetically related strains from being separated. However, we strongly recommend combining cgMLST with in silico serotyping to maintain backward compatibility with the current Shigella serotyping scheme. Strain selection and typing In total, 4187 Shigella reference strains and clinical isolates were studied (Supplementary Data 1 ). Two datasets were used. The first dataset – the “reference” dataset – consisted of 317 Shigella reference strains covering all the known serotypes – including provisional serotypes – from various geographic locations (53 countries on four continents) and time periods (1913 to 2019). These strains originated from the French National Reference Centre for E. coli , Shigella , and Salmonella (FNRC-ESS), Institut Pasteur, Paris, except for 11 strains belonging to provisional serotypes and provided by the Public Health Agency of Canada, Winnipeg, Canada; the Centers for Disease Control and Prevention, Atlanta, USA; the Tokyo Metropolitan Research Laboratory of Public Health, Tokyo, Japan; and the International Centre for Diarrhoeal Disease Research, Bangladesh, Dhaka. This “reference” dataset included 44 S. sonnei from four different lineages [33] , 16 S. dysenteriae type 1 (ref. [34] ) and 98 S. flexneri serotypes 1–5, X and Y belonging to the seven phylogenetic groups (PGs) described previously [2] , [5] . The second dataset – the “routine” dataset – consisted of 3870 clinical isolates received and sequenced by the FNRC-ESS between 2017 and 2020 in the framework of the French national surveillance programme for Shigella infections. This programme is based on a voluntary laboratory-based network consisting of ~1000 clinical laboratories located in mainland France and its overseas territories in South America, the Caribbean and Indian Ocean, which send ~1000–1200 Shigella isolates to the FNRC-ESS each year (only 600 in 2020, due to the COVID pandemic). This surveillance system has been estimated to detect 50–60% of laboratory-confirmed Shigella infections in France [35] . Between 2017 and 2020, 3942 clinical isolates were received and sequenced at the FNRC-ESS, and we included the 3870 genomes that passed the quality control criteria of EnteroBase. All these strains and isolates were thoroughly characterised with a panel of biochemical tests and serotyped by slide agglutination assays according to standard protocols, as previously described [36] . Additional typing sera against KIVI 162 and SH-105 were provided by the International Centre for Diarrhoeal Disease Research, and the Public Health Agency of Canada, respectively. DNA extraction and sequencing Total DNA was extracted with the Wizard Genomic DNA Kit (Promega, Madison, WI, USA), the Maxwell 16-cell DNA purification kit (Promega) or the MagNA Pure DNA isolation kit (Roche Molecular Systems, Indianapolis, IN, USA), in accordance with the manufacturer’s recommendations. The 4187 strains and isolates were sequenced with different Illumina platforms. FqCleanER version 3.0 ( https://gitlab.pasteur.fr/GIPhy/fqCleanER ) was used to eliminate adaptor sequences [37] , correct sequencing errors [38] and discard low-quality reads. Assemblies were generated with SPAdes [39] version 3.15. 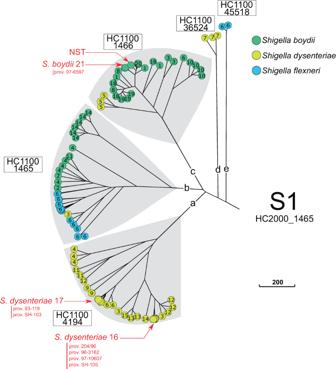Other studied genomes With the aim of capturing the broadest possible diversity of S higella populations, we searched the E. coli / Shigella database in EnteroBase [18] , and selected 81 additional Shigella genomes (“reference+” dataset) not originating from the Institut Pasteur (Supplementary Methods section “Other studied genomes”). We included 27 enteroinvasive E. coli (EIEC) and 68 E. coli strains from the E. coli reference (ECOR) collection (Supplementary Methods section “Other studied genomes”), to place our Shigella genomes in the phylogenetic context of the broader diversity of E. coli . We also used the closed PacBio sequences available for all Shigella serotypes and described by Kim and coworkers [40] , to study the genetic organisation of the rfb gene cluster or various operons described in the “Gene analyses” section. However, these closed genomes were not included in the cgMLST analysis, as they were not edited with short reads and the numerous indels in the homopolymers therefore altered the allelic distances (Supplementary Table 1 ). Characterisation of the O-antigen gene clusters The Shigella O-antigen biosynthetic gene ( rfb ) cluster was analysed after extraction of the region between the housekeeping genes galF (encoding UTP-glucose-1-phosphate uridylyltransferase) and gnd (encoding 6-phosphogluconate dehydrogenase), which are known to flank the rfb cluster [28] . Newly identified rfb clusters were annotated on the basis of a previously annotated closely matched E. coli cluster in the NCBI BLASTn nucleotide collection (nr/nt) database (100% coverage and at least 99% identity) or with ORFfinder ( https://www.ncbi.nlm.nih.gov/orffinder/ ) when no matching cluster was found in the NCBI BLAST database ( https://blast.ncbi.nlm.nih.gov/Blast.cgi ). Fig. 2: A NINJA NJ GrapeTree showing the population structure of theShigellaS1 cluster (HC2000_1465). This subtree is based on the tree shown in Fig.1. The tree nodes are colour-coded by serogroup. The numbers within nodes indicate the serotype. HC1100 designation is indicated next to each subcluster. Novel and provisional (prov.)Shigellaserotypes are also shown. NST non-serotypeable. The scale bar indicates the number of cgMLST allelic differences. The GenBank accession codes of all the Shigella rfb clusters are listed in Supplementary Table 2 . We also used three tools for in silico serotyping: SeroPred, the serotype prediction tool implemented in EnteroBase [18] , ShigaTyper [14] (using short reads), and ShigEiFinder [16] (using both short reads and assemblies). Phylogenetic analyses We used the Escherichia / Shigella cgMLST scheme (“cgMLST V1”) implemented in EnteroBase [18] to study our genomic datasets. This scheme is based on 2513 single-copy orthologous genes found in the soft-core genome of a representative set of Escherichia and Shigella genomes [18] . The cgMLST sequence types (cgSTs) consist of a combination of up to 2513 integers, each representing a sequence variant (allele) of a gene, accounting for missing data (gene missing, allele not called due to short-read misassemblies). Genetic distances between genomes were calculated from the number of shared cgMLST alleles. The cgMLST trees were inferred with the NINJA neighbour-joining algorithm, present in the “cgMLST V1+HierCC V1” scheme of EnteroBase. We visualised the cgMLST data with GrapeTree [41] . These bacterial genomes were also assigned to clusters at multiple levels of resolution, by a single-linkage hierarchical clustering pipeline (pHierCC), implemented in the “cgMLST V1+HierCC V1” scheme, and described in detail by Zhou and coworkers [19] . Each genome was assigned to 13 clusters – one for each level of resolution (HC0, HC2, HC5, HC10, HC20, HC50, HC100, HC200, HC400, HC1100, HC1500, HC2000 and HC2350) – with stable numbers. In EnteroBase, genomes equidistant from multiple clusters were assigned to the oldest cluster (i.e., with the smallest HC number) in order to ensure the long-term stability of the nomenclature. Genomes with >3% of missing data were also processed separately by pHierCC to minimise the impact of missing data on clustering [19] . We also performed cgSNV analysis to assess the phylogenetic relationships of 398 Shigella (317 from the “reference” dataset and 81 from the “reference+” dataset) and 95 E. coli (68 ECOR and 27 EIEC) strains. An Escherichia fergusonii genome (RHB19-C05, GenBank accession no. GCF_013892435.1) was used as an outgroup for the cgSNV analysis. The paired-end reads and simulated paired-end reads were mapped onto the reference genome of E. coli K12-MG1655 (GenBank accession no. NC_000913.3) with Snippy version 4.6 ( https://github.com/tseemann/snippy ). We used Snippy default settings, except–mincov 4–minfrac 0.75, to ensure consistency with previous work [34] . Gubbins [42] version 2.4.1 (default settings, except -f 30) was used to identify regions of recombination within the core genome alignment. Two alignments were used for phylogenetic inference, one of 92,688 SNVs (including recombinant sites) and a second alignment of 5129 SNVs (recombination removed). We generated maximum-likelihood (ML) phylogenetic trees with RAxML-NG [43] version 1.0.1 using the general time-reversible (GTR) model of nucleotide substitution with a gamma model of between-site heterogeneity rate (GTR+G) and 100 bootstrap iterations. The best-scoring ML tree of the 20 replicates was midpoint-rooted and visualised with interactive tree of life (iTOL) [44] version 6 ( https://itol.embl.de ). 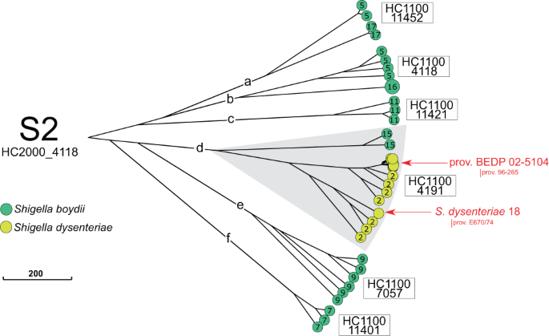A phylogenetic tree of rfb sequences was constructed with the sequences from 43 Shigella (Supplementary Table 2 ) and 196 E. coli strains from DebRoy and coworkers [28] . The Shigella rfb sequences were trimmed to ensure the same start and end points as for the E. coli rfb sequences from DebRoy and coworkers [28] . A sequence alignment was generated with MEGA X [45] version 10.2.1, using ClustalW with default settings. A ML phylogeny was created with RAxML-NG [43] version 1.0.1, using the GTR+G model and 100 bootstrap replicates. The ML tree with the best score of the 20 replicates was midpoint-rooted and visualised with iTOL [44] version 6 ( https://itol.embl.de ). Gene analyses The presence of the ipaH gene, a multicopy gene unique to Shigella and EIEC [46] , the presence and structure of the mannitol ( mtl ) [47] , raffinose ( raf ) [48] , and tryptophanase ( tna ) operons [49] and the type of the O-antigen gene cluster ( rfb ) were determined using SPAdes assemblies with NCBI BLASTn version 2.10.1 ( https://blast.ncbi.nlm.nih.gov/Blast.cgi ). Fig. 3: A NINJA NJ GrapeTree showing the population structure of theShigellaS2 cluster (HC2000_4118). This subtree is based on the tree shown in Fig.1. The tree nodes are colour-coded by serogroup. The numbers within nodes indicate the serotype. HC1100 designation is indicated next to each subcluster. Provisional (prov.)Shigellaserotypes are also shown. The scale bar indicates the number of cgMLST allelic differences. The target sequences are described in Supplementary Table 3 . Data collection The data were entered into an Excel (Microsoft) version 15.41 spreadsheet (Supplementary Data 1 ). Reporting summary Further information on research design is available in the Nature Research Reporting Summary linked to this article.